Synthetic optical holography for rapid nanoimaging Holography has paved the way for phase imaging in a variety of wide-field techniques, including electron, X-ray and optical microscopy. In scanning optical microscopy, however, the serial fashion of image acquisition seems to challenge a direct implementation of traditional holography. Here we introduce synthetic optical holography (SOH) for quantitative phase-resolved imaging in scanning optical microscopy. It uniquely combines fast phase imaging, technical simplicity and simultaneous operation at visible and infrared frequencies with a single reference arm. We demonstrate SOH with a scattering-type scanning near-field optical microscope (s-SNOM) where it enables reliable quantitative phase-resolved near-field imaging with unprecedented speed. We apply these capabilities to nanoscale, non-invasive and rapid screening of grain boundaries in CVD-grown graphene, by recording 65 kilopixel near-field images in 26 s and 2.3 megapixel images in 13 min. Beyond s-SNOM, the SOH concept could boost the implementation of holography in other scanning imaging applications such as confocal microscopy. Optical holography [1] , [2] , [3] , [4] , [5] is an imaging technique where the light scattered from an illuminated object is superposed with a reference wave as in Fig. 1a . The resulting interference pattern—the hologram—encodes the complex optical field scattered from an object within a single image. Digital wide-field holograms have revolutionized modern holography, allowing the computation of amplitude and phase images in real time [6] , [7] . The combination of speed and ease of implementation has established holography as a scientific tool for imaging as well as for metrology and product inspection [7] , [8] . The application potential of holography has triggered the development of digital holographic microscopy, a wide-field technique providing quantitative phase [9] , [10] , three-dimensional information [4] , [11] , [12] , [13] , numerical refocusing [4] , [14] , [15] and aberration correction [14] . 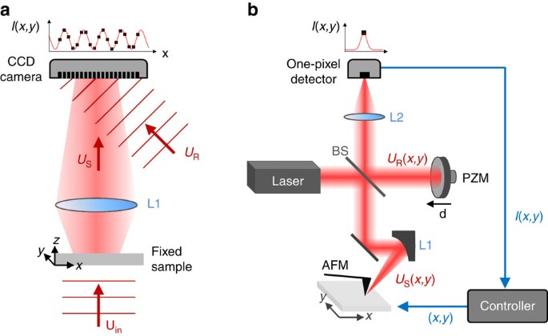Figure 1: Holography concepts. (a) Wide-field image-plane holography. (b) Synthetic optical holography (SOH) implemented in a scattering-type scanning near-field optical microscope (s-SNOM). AFM, atomic force microscope; BS, beam splitter; L1, L2, lenses; PZM, piezo-actuated mirror. Figure 1: Holography concepts. ( a ) Wide-field image-plane holography. ( b ) Synthetic optical holography (SOH) implemented in a scattering-type scanning near-field optical microscope (s-SNOM). AFM, atomic force microscope; BS, beam splitter; L1, L2, lenses; PZM, piezo-actuated mirror. Full size image In contrast to wide-field techniques, holography in confocal optical microscopy or scanning near-field optical microscopy is a widely unexplored terrain. This is surprising, as the mutual information between pixels (as in wide-field holograph) may allow for simplified phase contrast mapping in, for example, confocal optical microscopy, which offers superior contrast and spatial resolution for biological imaging. Similarly, scanning near-field optical microscopy based on infrared scattering at an atomic force microscope (AFM) tip (s-SNOM) [16] , [17] , [18] , [19] enables nanoscale resolved chemical, structural and conductivity mapping of nanocomposite materials [20] , [21] , [22] , [23] , [24] , [25] and biological matter [26] , [27] as well as plasmons in graphene [28] , [29] , [30] , [31] and metal nanostructures [32] , [33] , [34] , [35] . The main challenge of implementing holography is that these microscopy techniques usually employ point detectors while digital wide-field holography requires cameras ( Fig. 1a ). Holographic techniques have appeared in confocal microscopy using a camera instead of a point detector and only as a means to determine the phase at each position of the individual pixels separately, rather than encoding the phase across the whole image as in wide-field holography [36] , [37] . In the near-field, holography has been implemented with superoscillatory reference waves, that is, waves with spatial variation a few times faster than waves in free space. Superoscillatory waves were generated by total internal reflection at a prism face directly on the sample [38] , but at least two images are needed to determine phase and amplitude [39] . To determine the phase and amplitude in a single near-field hologram, hyperoscillatory reference waves, that is, waves with spatial variation hundreds of times faster than waves in free space, are required, but generation of such waves by total internal reflection requires a prism with unphysically large index of refraction. Thus, a truly holographic technique in which the complex field is encoded in a single image is yet to be achieved in scanning optical imaging. Here we introduce synthetic optical holography (SOH) based on synthetic reference waves (SRWs) [40] , [41] , [42] , [43] to enable holography in-phase-resolved s-SNOM for near-field imaging with significantly improved speed and simplified technology. We first describe and verify the SOH method with a well-know sample (dipole antenna), and demonstrate amplitude and phase imaging at visible and infrared frequencies simultaneously with a single reference arm. Having established SOH as a reliable and fast method for amplitude and phase-resolved near-field imaging, we demonstrate rapid infrared nanoimaging and application of SOH for large-area near-field mapping of chemical vapour deposition (CVD)-grown graphene. The graphene images reveal a network of grain boundaries owing to the large reflection of tip-induced graphene plasmons [28] , [29] at grain boundaries [31] . The general concept of SOH We introduce SOH as a general concept that aims at rapid, technically simple and quantitative phase imaging in scanning optical microscopy. In SOH, the field U S ( r ) obtained by local probing the sample at position r is superposed at a one-pixel detector with a reference field . Examples for local probes include a diffraction limited laser focus or an optical near-field probe. While scanning the sample or the local probe, the phase of the reference field ϕ R ( r ) is slowly varied to encode amplitude and phase of U S ( r ) across the image rather than varying the reference phase ϕ R at each position r as done in interferometric methods. In the fashion of wide-field holography, we thus take advantage of the mutual information between the pixels. Recording the detector signal I ( r ) pixel-by-pixel, we obtain a synthetic image-plane hologram of the sample, Equation (1) is the generic expression of a synthetic hologram, where U S could be any field scattered, reflected or transmitted in a scanning microscopic set-up. For a linearly-in-time changing reference phase ϕ R , equation (1) is identical to a wide-field hologram, from which amplitude and phase of U S can be recovered by standard reconstruction methods. In contrast to wide-field holography, the reference field U R ( r ) is generated sequentially, and thus is termed SRW. In the following, we describe and demonstrate the SOH concept for s-SNOM. The implementation of SOH in s-SNOM In s-SNOM, the sample is illuminated with monochromatic, coherent light and the light scattered from the apex of a vertically oscillating AFM tip is recorded while the sample is scanned. To measure the local near field scattered by the tip, U NF , background fields U B have to be suppressed. To that end, the scattered field U S = U NF + U B is combined with a reference field U R , and the detector intensity I is demodulated at the n th harmonic of the tip oscillation frequency Ω to obtain the demodulated intensity I n (see Supplementary Notes 1 and 2 ). In current variants of s-SNOM, the reference field has to be varied at each pixel (for example, frequency shifted or phase modulated), to interferometrically obtain from I n (i) background-free and (ii) amplitude and phase-resolved near-field images for n >2 (refs 44 , 45 ). To that end, technologically challenging techniques have been implemented, including heterodyne [44] , [46] , [47] , [48] , pseudo-heterodyne [45] or phase shifting [49] , [50] interferometry. In Fig. 1b we illustrate the implementation of SOH in s-SNOM. At each position r =( x , y ), the scattered field from the tip is superposed at the detector with a reference field . The reference phase ϕ R ( r )=2 π ·2 d ( r )/ λ is controlled by the position d ( r ) of a piezo-actuated reference mirror. While the tip is rapidly scanned over the sample, the reference mirror is slowly translated, yielding a single (quasi-constant) reference phase at each pixel. To obtain a synthetic near-field hologram, the n th order demodulated detector signal, I n ( r ), is recorded, rather than I ( r ): The terms in equation (2) represent the coefficients of the time-harmonic components of the scattered field, which for n >2 yield the background-free near-field signal (see Supplementary Notes 1 and 2 ). By applying a linear mirror translation at constant velocity v R , we generate a SRW analogous to a plane reference wave in off-axis wide-field holography, (see Methods). Thus, amplitude A S, n and phase ϕ S, n of the near-field signal U S, n ( r ) can be reconstructed from the near-field hologram I n ( r ) using standard Fourier transform (FT) filtering. The FT of the near-field hologram I n ( r ) reads where the tilde indicates FT with respect to position. C n is the n th order demodulation of the autocorrelation, that is, the FT of . The direct term and its conjugate are shifted by − k || and k || , respectively. By simple filtering, the direct term is isolated from the other terms and, performing an inverse FT, we obtain for n >2, background-free near-field optical amplitude and phase images, A S, n and ϕ S, n , as we illustrate below in Fig. 2 . 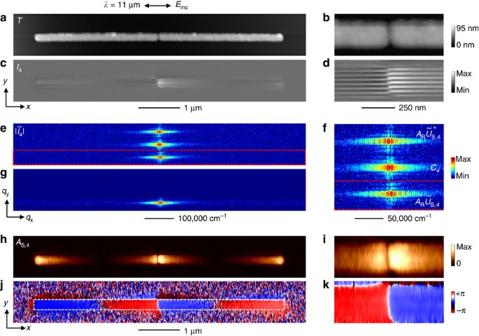Figure 2: Experimental demonstration and verification of the SOH concept by near-field imaging of an infrared antenna. (a) TopographyTof the antenna, showing two longitudinally aligned Au rods of 2.9 μm length and 50 nm height, separated by a 50-nm gap and supported on a CaF2substrate. (b) TopographyT, zoom of the gap region of the antenna. (c) HologramI4(r), yielding 700 × 100 pixels. Topography and hologram have been acquired simultaneously in 14 min. (d) HologramI4(r), zoom of the gap region. (e) Magnitude of Fourier transform,, ofI4(r). (f) Zoom of centre part ofshowing three peaks corresponding to the conjugate term, autocorrelation termC4and the direct term(top to bottom). (g) Filtered FT by applying a Hamming window according to the red dashed box ine. (h,j) Reconstructed amplitude and phase images,AS,4(r) andϕS,4(r), obtained by recentering ofgand subsequent inverse FT. (i,k) Zoom of the gap region showingAS,4(r) andϕS,4(r). Figure 2: Experimental demonstration and verification of the SOH concept by near-field imaging of an infrared antenna. ( a ) Topography T of the antenna, showing two longitudinally aligned Au rods of 2.9 μm length and 50 nm height, separated by a 50-nm gap and supported on a CaF 2 substrate. ( b ) Topography T , zoom of the gap region of the antenna. ( c ) Hologram I 4 ( r ), yielding 700 × 100 pixels. Topography and hologram have been acquired simultaneously in 14 min. ( d ) Hologram I 4 ( r ), zoom of the gap region. ( e ) Magnitude of Fourier transform, , of I 4 ( r ). ( f ) Zoom of centre part of showing three peaks corresponding to the conjugate term , autocorrelation term C 4 and the direct term (top to bottom). ( g ) Filtered FT by applying a Hamming window according to the red dashed box in e . ( h , j ) Reconstructed amplitude and phase images, A S,4 ( r ) and ϕ S,4 ( r ), obtained by recentering of g and subsequent inverse FT. ( i , k ) Zoom of the gap region showing A S,4 ( r ) and ϕ S,4 ( r ). Full size image We note that filtering the direct term effectively removes the multiplicative background term that is contained in the autocorrelation term C n . The multiplicative background term, , is caused by interference between near-field and background components contained in the scattered field (see Supplementary Note 2 ) and may produce artifacts in the near-field images. In conventional s-SNOM, it is typically suppressed by heterodyne or pseudo-heterodyne detection of the tip-scattered light [44] , [45] , [46] , [47] , [48] , [51] . Suppression of the multiplicative background with SOH thus offers reliable amplitude and phase mapping, while also being substantially technically simplified compared with methods where amplitude and phase are measured individually at each pixel. Verification of SOH with a plasmonic nanoantenna We demonstrate holographic near-field amplitude and phase mapping at wavelength λ =11 μm with a linear infrared dipole antenna exhibiting a well-defined amplitude and phase contrast on the nanometre scale [34] . We employ a dielectric tip to scatter the near fields of the antenna [34] , [35] . To map the vertical near-field component, the p -polarized scattered light is recorded [52] . Figure 2a,c shows topography and the simultaneously acquired hologram I n =4 of the antenna, which exhibits the typical fringe pattern of an image-plane hologram. The signal maxima appear approximately every 30 nm, demonstrating the synthesis of a hyperoscillatory reference wave with a virtual wave vector k || of magnitude 367 larger than the free space wavenumber (see Methods), a key to extreme subwavelength-scale holography. To reconstruct the near-field U S,4 of the sample, we take the FT of the hologram ( Fig. 2e ). We clearly see the autocorrelation term C 4 in the centre of the FT, as well as the terms and , which have separated into the lower and upper halves of the FT plane, respectively. To isolate the direct term , we apply a window to the FT as indicated by the dashed red box in Fig. 2e and obtain the filtered FT ( Fig. 2g ). Shifting the result to the centre of the FT plane and taking the inverse FT, we reconstruct the near-field amplitude and phase images of the antenna, A S,4 ( r ) and ϕ S,4 ( r ) ( Fig. 2h,j ). The observed near-field distribution reveals the expected fundamental dipolar mode of the antenna, characterized by strong fields at the rod extremities that oscillate 180° out-of-phase [34] , in good agreement with the numerically calculated near-field distribution (see Supplementary Fig. 1 ). Multicolour SOH In Fig. 3 we show that SOH allows for phase imaging at widely different frequencies with a single reference arm and simultaneously. To this end, we superimpose the beams of a HeNe laser ( λ 1 =633 nm) and a quantum cascade laser ( λ 2 =5.75 μm) and performed SOH s-SNOM mapping of an Au film on Si, a typical s-SNOM test sample with a well-defined contrast ( Fig. 3a ). The tip-scattered light is interfered with the reference beams and detected by a visible detector D1 and an infrared detector D2, the latter two providing the spectral separation. Intriguingly, only a single, linear-moving reference mirror is needed to generate synthetic holograms for both wavelengths (see Methods). By recording the detector signals while scanning the sample, we obtain a visible and an infrared hologram, I 3 (D1) and I 3 (D2) ( Fig. 3c,d ). Reconstruction of the individual holograms yields near-field amplitude and phase images. While no phase contrast is observed at the infrared wavelength λ 2 =5.75 μm, at λ 1 =633 μm a phase contrast of ϕ 3 (Au)− ϕ 3 (Si)=25° is found owing to the plasmon-resonant coupling between the near-field probe and the Au film [44] . Note that the wave-like contrast on the Au film at λ 1 =633 nm, we attribute to propagating plasmons launched at the edge of the Au film [53] . 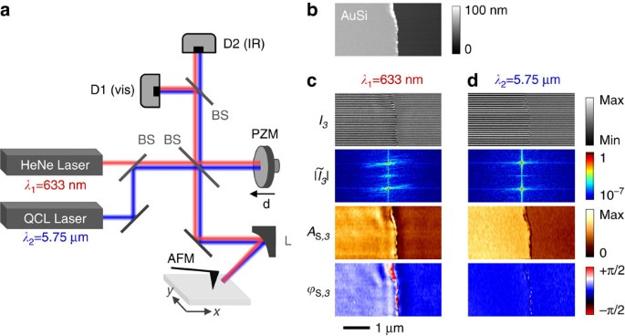Figure 3: Amplitude and phase imaging simultaneously at a visible and an infrared wavelength with a single reference arm. (a) Simplified schematic of a set-up for holographic s-SNOM imaging at two wavelengths with two detectors. AFM, atomic force microscope; BS, beam splitter (uncoated ZnSe window); L, lens, PZM, piezo-actuated mirror; D1, visible detector; D2, infrared detector. (b) Topography image of an Au-Si edge test sample. (c,d) Near-field hologramsI3(D1) andI3(D2) and their FTsandobtained by recording the signals from detectors D1 and D2. Reconstructed amplitude and phase images,AS,3andϕS,3, at wavelengthsλ1=633 nm andλ2=5.75 μm. Figure 3: Amplitude and phase imaging simultaneously at a visible and an infrared wavelength with a single reference arm. ( a ) Simplified schematic of a set-up for holographic s-SNOM imaging at two wavelengths with two detectors. AFM, atomic force microscope; BS, beam splitter (uncoated ZnSe window); L, lens, PZM, piezo-actuated mirror; D1, visible detector; D2, infrared detector. ( b ) Topography image of an Au-Si edge test sample. ( c , d ) Near-field holograms I 3 (D1) and I 3 (D2) and their FTs and obtained by recording the signals from detectors D1 and D2. Reconstructed amplitude and phase images, A S,3 and ϕ S,3 , at wavelengths λ 1 =633 nm and λ 2 =5.75 μm. Full size image Application for rapid screening of CVD-grown graphene SOH allows for rapid amplitude and phase-resolved near-field imaging, which in the following is applied for non-invasive large-area screening of graphene grain boundaries with nanometre-scale precision. Recently, it has been shown that the strongly concentrated near fields at the apex of a metal s-SNOM tip can launch plasmon polaritons—coupled excitations of photons and charge carriers—in graphene layers. These waves are partially reflected at graphene edges, gaps and defects [28] , [29] , [30] , [31] causing interference between the local field at the tip apex and the reflected plasmon waves. Recording the tip-scattered field reveals the plasmon interference pattern that contains valuable information on the plasmon properties such as plasmon wavelength and propagation losses [31] . In CVD-grown graphene layers, plasmons are strongly reflected at grain boundaries, yielding bright interference fringes to either side of the boundary. The quantitative analysis of the plasmon interference pattern provides interesting insights into the electronic properties of graphene, such as an increased carrier concentration and reduced mobility near the grain boundaries [31] . With the growing interest in CVD graphene, both the non-invasive and rapid mapping of grain boundaries—which diminish the mechanical and electrical properties of graphene [31] , [54] , [55] —will benefit the optimization of growth processes and quality control. We demonstrate rapid large-scale screening of graphene boundaries in Fig. 4 by presenting infrared near-field images of a 21 × 21 μm 2 area of CVD-grown graphene. Applying SOH, the 2.3 megapixel image could be acquired in only 13 min. We note that with state-of-the art commercial pseudoheterodyne detection (Neaspec PMDK-2 module), the image acquisition would take 8 h, as for technical reasons the minimum integration time per pixel is 6.5 ms. The topography image shows dirt particles and graphene wrinkles ( Fig. 4a ), while the infrared amplitude and phase images ( Fig. 4c,d ) reconstructed from the recorded hologram ( Fig. 4b ) and its FT ( Fig. 4b , inset) clearly exhibit a network of twin fringes. As discussed above and in more detail in ref. 31 , the twin fringes ( A S,3 in Fig. 4e ) reveal grain boundaries in the graphene layer. Depicting the boundaries by black lines in Fig. 4f (see Methods), we recover the network of grain boundaries that clearly resembles the results obtained from transmission electron microscopic images [55] , [56] . SOH s-SNOM thus offers the advantage of non-invasive, rapid screening of graphene layers on substrates, avoiding radiation damage potentially introduced by electron exposure. 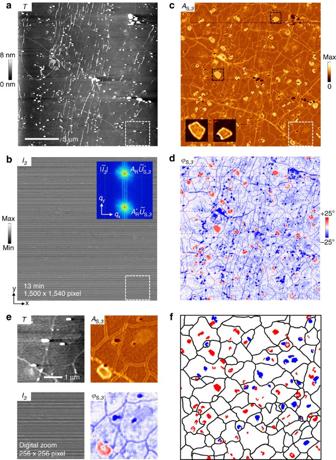Figure 4: Large-scale non-invasive quality screening of CVD-grown graphene with SOH s-SNOM. (a) TopographyT. (b) HologramI3(r) acquired atλ=10.55 μm. Both topographyTand hologramI3(r) (21 × 21 μm2, 1,500 × 1,540 pixel) were acquired simultaneously in 13 min, scanning the sample at a velocity of 88 μm s−1and recording the infrared detector signal at a pixel rate of 6,600 Hz. (c) Infrared amplitudeAS,3(r). The insets show contrast-enhanced digital zooms on two multilayer graphene patches marked by the black dashed boxes, revealing plasmon interference patterns. (d) Infrared phaseϕS,3(r). (e) Digital zooms (3.5 × 3.5 μm2, 256 × 256 pixel) of the area marked by the white dashed boxes ina–d. (f) Map of grain boundaries (black lines), plasmon-active multilayers (red) and plasmon-inactive multilayers (blue). Figure 4: Large-scale non-invasive quality screening of CVD-grown graphene with SOH s-SNOM. ( a ) Topography T . ( b ) Hologram I 3 ( r ) acquired at λ =10.55 μm. Both topography T and hologram I 3 ( r ) (21 × 21 μm 2 , 1,500 × 1,540 pixel) were acquired simultaneously in 13 min, scanning the sample at a velocity of 88 μm s −1 and recording the infrared detector signal at a pixel rate of 6,600 Hz. ( c ) Infrared amplitude A S,3 ( r ). The insets show contrast-enhanced digital zooms on two multilayer graphene patches marked by the black dashed boxes, revealing plasmon interference patterns. ( d ) Infrared phase ϕ S,3 ( r ). ( e ) Digital zooms (3.5 × 3.5 μm 2 , 256 × 256 pixel) of the area marked by the white dashed boxes in a – d . ( f ) Map of grain boundaries (black lines), plasmon-active multilayers (red) and plasmon-inactive multilayers (blue). Full size image The infrared near-field images also show graphene multilayer islands exhibiting either a bright or a dark infrared contrast. We attribute this observation to different plasmonic properties. We emphasize the bright (red) and dark (blue) multilayer islands in the map in Fig. 4f . Further studies are required to clarify the contrast variation between different multilayers, which, however, would go beyond the scope of this paper. We conclude that the rich variety of information in large-scale near-field phase and amplitude images clearly holds great potential for process and quality control in graphene production. SOH also provides near-field phase images ( Fig. 4d and ϕ S,3 in Fig. 4e ). Interestingly, the grain boundaries appear only as a single fringe in the phase image, which is located between the amplitude fringes. As near-field phase images of graphene plasmon interference have not been reported yet, we briefly discuss their significance in Fig. 5 . To this end, we take high-resolution near-field images of a graphene grain boundary ( Fig. 5a ) and extract a line profile perpendicular to the grain boundary, yielding the measured near-field amplitude A S,3 ( d ) and phase ϕ S,3 ( d ) as a function of the distance d of the tip from the grain boundary ( Fig. 5b ). While in amplitude we find the typical profile of a twin fringe in accordance to ref. 31 , the phase profile shows an oscillatory behaviour similar to the amplitude signal. To understand the phase contrast, we plot the left half of the line profile in the complex plane ( Fig. 5c ). The data have been normalized to the near-field signal on graphene far from the grain boundaries (marked by ‘R’ in Fig. 5a ). At this point, the near-field signal represents the initial local near field below the tip apex, E i , governed by the near-field interaction between the tip, substrate and graphene, without the influence of reflected plasmons [31] . Near the grain boundary, the field of the reflected plasmons E p ( d ) significantly adds to the initial local field E i ; thus, a total field E t ( d )= E p ( d )+ E i is measured at the tip. As the tip approaches the grain boundary (marked by ‘GB’), we observe that the field vector E p ( d ) evolves in a spiral manner relative to E i , that is, the phase ϕ p of the plasmon field steadily increases for more than 360°. The complex representation thus provides direct experimental evidence of the propagating nature of the graphene plasmons. For a brief analysis, we fit the model for plasmon interference fringes from ref. 31 to our complex-valued data in Fig. 5c . 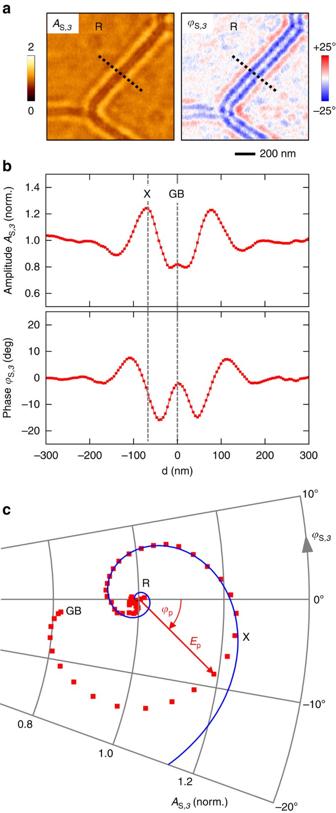Figure 5: Amplitude and phase profiles of plasmon interferometry at a graphene grain boundary. (a) Near-field amplitude and phase images,AS,3andϕS,3, of a graphene grain boundary (1.3 × 1.3 μm2, 256 × 256 pixel, 26 s by applying SOH,λ=10.59 μm wavelength). (b) Line profile in amplitude and phase taken along the dashed line ina. (c) Complex plot of the line profile (dots, experimental data; line, fit). The data have been normalized to an area marked by ‘R’ ina. GB, grain boundary; X, point at a distanced=75 nm to GB (see text), R, reference area for normalizing the near-field signals. The model describes the tip-launched plasmon waves by attenuated two-dimensional cylindrical waves, yielding a total field E t ( d ) at the tip Figure 5: Amplitude and phase profiles of plasmon interferometry at a graphene grain boundary. ( a ) Near-field amplitude and phase images, A S,3 and ϕ S,3 , of a graphene grain boundary (1.3 × 1.3 μm 2 , 256 × 256 pixel, 26 s by applying SOH, λ =10.59 μm wavelength). ( b ) Line profile in amplitude and phase taken along the dashed line in a . ( c ) Complex plot of the line profile (dots, experimental data; line, fit). The data have been normalized to an area marked by ‘R’ in a . GB, grain boundary; X, point at a distance d =75 nm to GB (see text), R, reference area for normalizing the near-field signals. Full size image where q p is the local plasmon momentum, δ the plasmon phase shift on reflection off the grain boundary and C 0 and | r (0)| are constants. We find that equation (4) produces a good fit to our data when only the inner part of the spiral curve is considered, that is, data recorded up to a distance d =75 nm (mark ‘X’) to ‘GB’. We obtain a plasmon wavelength of λ p =286 nm, a damping rate of γ p =0.26 and a phase shift δ =155°, similar to ref. 31 . In the outer part of the spiral curve, however, the fit (blue curve) predicts a steadily increasing magnitude | E p | while our data indicate a saturation of | E p | (red dots). This deviation we explain by a local modification of the electronic properties (increased Fermi energy and a reduced DC conductivity) of graphene near the grain boundary, as has been discussed in detail in ref. 31 . In the future, exploring and fitting both amplitude and phase profiles might benefit the quantitative analysis of plasmon interference phenomena in graphene layers, which, however, would go beyond the scope of this paper. Comparison of SOH with interferometric methods In Fig. 6a–d we compare the performance of SOH s-SNOM with conventional s-SNOM. To that end, we have chosen the graphene grain boundary of Fig. 5 as a test object, providing a defined near-field amplitude and phase contrast. Employing different detection methods, we recorded near-field images in 26 s (10 Hz line rate) under the same conditions (see Methods). For further comparison, we show in Fig. 6e s-SNOM images taken with a state-of-the-art commercial pseudoheterodyne module (same as used in refs 28 , 29 , 30 , 31 for graphene plasmon mapping). 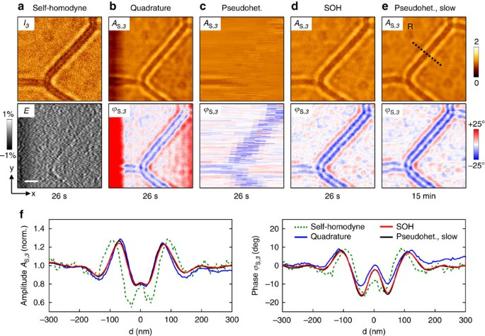Figure 6: Comparison of SOH with interferometric methods by rapidly imaging a graphene boundary. All images are 256 × 256 pixel and were recorded atλ=10.59 μm and in 26 s. (a) Top: Self-homodyne intensity image. Bottom: AFM error signalEnormalized to the lock-in amplitude of the cantilever deflection signal. Scale bar, 200 nm. (b) Quadrature homodyne detection. (c) Pseudoheterodyne detection. (d) SOH. (e) Reference images recorded with state-of-the-art commercial pseudoheterodyne detection at a standard imaging time of 14 min. The amplitude and phase signals ina–e,AS,3andϕS,3have been normalized to a region far from the grain boundaries indicated by the mark ‘R’. (f) Line profiles taken from the images (a,b,d,e) along the path marked by the dashed line ine, averaged over a width of 400 nm (80 lines). Figure 6: Comparison of SOH with interferometric methods by rapidly imaging a graphene boundary. All images are 256 × 256 pixel and were recorded at λ =10.59 μm and in 26 s. ( a ) Top: Self-homodyne intensity image. Bottom: AFM error signal E normalized to the lock-in amplitude of the cantilever deflection signal. Scale bar, 200 nm. ( b ) Quadrature homodyne detection. ( c ) Pseudoheterodyne detection. ( d ) SOH. ( e ) Reference images recorded with state-of-the-art commercial pseudoheterodyne detection at a standard imaging time of 14 min. The amplitude and phase signals in a – e , A S,3 and ϕ S,3 have been normalized to a region far from the grain boundaries indicated by the mark ‘R’. ( f ) Line profiles taken from the images ( a , b , d , e ) along the path marked by the dashed line in e , averaged over a width of 400 nm (80 lines). Full size image In pseudoheterodyne (PSH) s-SNOM [45] , near-field amplitude and phase imaging is achieved by oscillating the reference mirror at a frequency M with amplitude 0.21 λ (for technical reasons, M is typically between 100 and 500 Hz). The detector signal is demodulated at n Ω+ M and n Ω+2 M , yielding two signals from which the near-field amplitude and phase are calculated online. Figure 6e shows 256 × 256 pixel amplitude and phase images, which were recorded simultaneously in a typical time of 14 min. Analogous to Fig. 5 , we observe twin fringes in the amplitude and phase images. In the following, these images serve as reliable reference. We then imaged the grain boundary in 26 s by employing self-homodyne (SH) detection [17] , [18] , [57] , where the scattered field is detected and demodulated without the interferometer ( Fig. 6a ). The imaging speed in this technique is not limited by the interferometer. However, only an intensity image I n ≈| U NF, n || U B,0 |cos( ϕ NF, n − ϕ B,0 ) can be recorded, which yields the interference between the near-field U NF and background U B,0 contribution in the scattered field U S . Although this intensity image exhibits a similar contrast as in Fig. 6e , the image contrast depends on the uncontrolled and unknown phase difference between near-field and background contribution, ϕ NF, n − ϕ B,0 , which generally does not allow for reliable near-field imaging [45] , [51] , [58] . Indeed, the intensity line profile across the grain boundary (dashed green curves) shown in Fig. 6f does neither fit the amplitude nor phase profile (black curves) obtained from the reference images shown in Fig. 6e . Next, we imaged the grain boundary with the quadrature homodyne (QH) method [32] , [33] , [59] , where the interference of the tip-scattered light with the external reference beam is recorded ( Fig. 6b ). To obtain both amplitude and phase, the detector signal at each pixel is measured at two different mirror positions, yielding an in-phase and out-of-phase signal from which amplitude and phase can be calculated [59] . We implemented the quadrature method by recording the forward scan of each line at a mirror position d and the backward scan of the same line at a mirror position d + λ /8. The amplitude and phase images show a similar qualitative contrast as observed in Fig. 6e . The profiles across the grain boundary (blue curves in Fig. 6f ), however, show quantitative discrepancies compared with the line profiles obtained from Fig. 6e (black curves in Fig. 6f ), particularly in the phase. We attribute them to the interference of background and near-field contributions (multiplicative background, as explained before), which cannot be suppressed by the quadrature method [45] , [51] . Furthermore, the left side of the phase image is distorted (red vertical stripe) and exhibits a slight gradient from left to right. These artifacts are caused by the required abrupt change of the mirror position at the beginning of each line that the piezo actuator driving the reference mirror is unable to perform instantly because of its inertia. The finite response time of the piezo actuator (measured to be 20 ms in our closed-loop system, see Methods) becomes a speed limitation for the quadrature method, particularly when fast scanning at line rates ⩾ 10 Hz. The amplitude and phase images obtained by pseudoheterodyne imaging in 26 s are shown in Fig. 6c . Both images are blurred, as the integration time of the employed commercial PSH module cannot be shorter than 6.5 ms for technical reasons (see below). Figure 6d shows the results obtained by SOH s-SNOM (same data as shown in Fig. 5a ). Both amplitude and phase images are in excellent quantitative agreement with Fig. 6e , which can be appreciated by comparing line profiles across the grain boundary (red curves in Fig. 6f ) with line profiles obtained from Fig. 6e (black curves in Fig. 6f ). Figure 6 clearly demonstrates the advantages of SOH. Compared with SH detection ( Fig. 6a ), SOH increases the signal-to-noise ratio (owing to I SOH, n = U NF, n U R > I SH, n ≈ U NF, n U B,0 because of | U R |>| U B |), yields both amplitude and phase images and avoids artefacts caused by the unknown phase difference between U NF, n and U B,0 . Compared with QH detection ( Fig. 6b ), SOH fully suppresses the multiplicative background term, , which in QH can be a cause of artifacts. Further, the relatively slow mirror movement in SOH avoids the artefacts caused by the abrupt mirror movements required in QH. The signal-to-noise ratio is similar between QH and SOH. Compared with PSH detection, SOH offers the advantage of faster data acquisition. We note that increasing the acquisition speed in PSH in principle is possible. However, high-frequency mirror vibration with large amplitudes of several micrometres bear technical problems, such as increased mechanical noise, possible mirror flexing and nonlinearities in the mirror vibration. Further, multicolour imaging, that is, amplitude and phase imaging at different illumination frequencies ( Fig. 3 ) is not possible with PSH. Regarding the signal-to-noise ratio, a direct comparison between SOH and PSH is not possible because of the lack of reasonable image contrast. However, it can be expected that the signal-to-noise is better in SOH, as in PSH the detector intensity is distributed over several sidebands, which are not involved in the data processing [45] . An alternative detection method for phase-resolved s-SNOM is heterodyne interferometry (HI) [44] , [46] , [47] , [48] . As it uses acousto-optical modulators to frequency shift the reference beam, HI allows for fast data acquisition and suppression of the multiplicative background. However, sophisticated synchronization between tip oscillation and frequency shift of the reference beam is required, which makes HI technically challenging to implement. Moreover, the acousto-optical modulator limits the applicable spectral range of HI, and in fact HI has not been demonstrated yet for phase-resolved s-SNOM at mid-infrared frequencies. SOH solves these problems because it only requires a linearly moving reference mirror. No synchronization between tip oscillation and mirror movement is needed, which makes SOH technically easy to implement. Most intriguingly, SOH allows for operation at visible and infrared frequencies with a single reference arm, even simultaneously. Note that the imaging speed in SOH s-SNOM is currently limited by the following two factors: the signal-to-noise ratio of the near-field signal and the scanning speed of the AFM. In Fig. 6 , our home-built AFM was operated near its maximum speed, which is limited by the responsiveness of the sample scanner (Physikinstrumente PI-517) and the AFM feedback for tip-sample distance control. The AFM error signal image ( Fig. 6a , bottom), simultaneously recorded to the near-field images shown in Fig. 6d , confirms that the variation of the tip oscillation amplitude was <0.4% (root mean squared), which lets us exclude mechanically induced near-field contrasts (artefacts). Assuming near-field signals with sufficiently large signal-to-noise ratio, faster imaging or imaging of samples with large topography would be possible with SOH s-SNOM, but would require the use of fast-scanning AFM technologies [60] , [61] . We furthermore note that SOH might not be applied to imaging an object with low resolution, for example, where an object appears as few individual pixels in the image. In the low resolution case, the object’s bandwidth can easily become very large, which results in an overlap of the direct and conjugate term in the FT space. In this case, the resolution needs to be increased by, for example, acquiring an image with more pixels until separation between direct and conjugate terms is achieved. SOH opens new horizons in holography and scanning microscopy far beyond the near-field imaging demonstrated here. Confocal microscopy has shown promise as a tool for high-resolution cellular imaging with important applications in neuroimaging [62] , but fluorescent dyes are often needed to improve contrast. Quantitative phase imaging could be an alternative, intrinsic contrast mechanism for cellular imaging, even in reflection [63] . SOH could simplify phase imaging in confocal systems to achieve fast, high-contrast cellular and subcellular contrast with no dyes or stains. Moreover, SRWs with arbitrary phase patterns, as well as super- and hyperoscillatory SRWs are easily generated and could be made into Haddemard masks or random basis functions used to implement compressive holography [64] , which has recently shown great potential in the imaging of sparse objects from minimal data sets. SOH offers particular advantages in the mid-infrared and THz spectral range, where scanning techniques and point detectors dominate imaging and microscopy. It could also be applied for holographic chemical mapping exploiting molecular vibrational absorption in the sample. The signal enhancement coming along with holographic detection could also benefit the development of highly sensitive infrared and THz scanners for security screening and quality control. SOH s-SNOM The s-SNOM used in this work is based on an AFM where a cantilevered tip acts as a near-field probe. The tip is illuminated at infrared wavelengths with a monochromatic, focused beam of a grating tunable CO 2 laser ( Fig. 1b ). The light scattered from the tip is collected with a parabolic mirror and superposed on the one-pixel detector with a synthetic reference wave (SRW). To suppress background contributions, the tip is vibrated at a frequency Ω=250 kHz (as in tapping mode AFM) and the detector signal is demodulated at frequencies 3 Ω and 4 Ω. In Figs 2 and 4 , the reference mirror is moved by a linear piezo stage with 100 μm travel (Physikinstrumente, model P-611). When the limit of the travel range is reached, the piezo is quickly retracted to the starting position and the linear translation is continued. This, yet not optimized, procedure yields minor artefacts in the images in Fig. 4 (visible as black or dashed horizontal lines). Operation in closed-loop mode compensates nonlinearity, hysteresis and creep of the piezo stage sufficiently well to enable the precise generation of SRWs even at visible frequencies. In Figs 3 , 5 and 6 , long-travel linear piezo stages with 1,500 and 800 μm range were employed (Physikinstrumente, models PiHera PI-629 and PI-628), which do not require quick piezo retracts during image acquisitions for standard image sizes. Using metal-coated tips (as in Figs 3 , 4 , 5 , 6 ), the illuminating light is converted into strongly concentrated near fields at the tip apex (nanofocus), which provides a means for localized excitation of molecule vibrations, plasmons or phonons at the sample surface. Recording of the scattered light thus allows for nanoscale mapping of the local chemical composition, conductivity or structural properties [16] , [20] , [21] , [25] . s-SNOM can also be used for imaging the near-field distribution of photonic nanostructures. In this particular application ( Fig. 2 ), a dielectric tip is employed to scatter the near-fields at the sample surface [34] , [35] . Fast sample scanning at velocities of v x =88 μm s −1 in Fig. 4 and v x =26 μm s −1 in Figs 5 , 6 was achieved by operating the AFM with a scan controller ‘NanoWizard’ from the company JPK with a time constant for the integrator of 200 Hz, a proportional gain of 0.04 and with the set point at ~80% of the free tapping amplitude of 190 nm in Fig. 4 and 150 nm in Figs 5 , 6 . Demodulation of the infrared detector sample was performed with pixel rates of 6,600 Hz in Fig. 4 and 5,100 Hz in Figs 5 , 6 . Sufficient signal-to-noise ratio was achieved by illuminating the tip with a CO 2 laser beam of ~20 mW in Fig. 4 and 6 mW power in Figs. 5 . Under such conditions, we expect even faster image recording by combining SOH with fast-scan AFM technology. In case of a low infrared signal-to-noise ratio (which occurs, for example, when weak laser sources are used or when low-dielectric samples are imaged), longer integration times may be required, which may then become the limiting factor for the imaging speed. Synthesis of a plane wave reference wave By translating linearly the reference mirror at velocity v R , a linearly-in-time changing reference phase is generated according to ϕ ( t )= φt + ϕ 0 where ϕ 0 is the reference phase at time t =0. The angular frequency φ is dependent on the wavelength λ and v R according to φ =2 π ·2 v R / λ where the extra factor of two accounts for the round trip in the reference arm. We assume that the tip is scanned along the principal directions of a Cartesian system, moving rapidly in the x direction such that x = v x t and that after travelling the total scan length X , it returns at the same speed and moves one step, Δ y , in the y direction. The effective velocity in the y direction is then v y = v x Δ y /(2 X ). The phase of the reference may thus be rewritten as a function of position, ϕ R ( r )= k || . r + ϕ 0 . Thus, the virtual wave vector k || =( k x , k y ) is given by k x = φ / v x , and k y = φ / v y =2 Xk x /Δ y =2 Xφ /( v x Δ y ). For the example of the dipole antenna, the hologram shown in Fig. 2a exhibits a virtual wave vector of k || ≈ k y ≈367 k 0 that mainly points in the y direction. The slow but continuous translation of the reference mirror also generates a small component in x direction, which we can calculate according to the above equations k x = v y / v x · k y =Δ y /(2 X )· k y ≈0.26 k 0 with Δ y =10 nm and X =7 μm. The value of k y =367 k 0 has been chosen such that the three terms (direct term , conjugate term and the autocorrelation term C n ) do not overlap in the FT. As in wide-field holography, only one component of the reference wave vector needs to be sufficiently large to separate the three terms. The spatial resolution of the reconstructed images is set by the choice of the filter applied to the FT of the hologram. The conjugate term and the autocorrelation term can be removed by making the filter bandwidth narrow in y direction, while the full bandwidth is allowed in x direction, as indicated by the red dashed box in Fig. 2b . Thus, the resolution is reduced by a factor of about 2 in the y direction, while the full resolution is maintained in x direction. Note that in the presented phase images in Figs 3 , 4 , 5 , slow phase fluctuations of the interferometer during the imaging process were removed in a post-process by line-wise subtraction of an average phase value. In the two-wavelength case presented in Fig. 3 , a slightly different scheme for the generation of SRWs was employed where the reference mirror was translated stepwise by Δ d =0.708 μm at the beginning of each line, although this was not a requirement in Fig. 3 and a linear motion of the reference mirror could have been applied as well. For the infrared wavelength λ 2 =5.75 μm, this translation corresponds to a phase step of Δ ϕ 2 =2 π ·2Δ d / λ 2 =1.547=0.49 π for each line. In case of the visible wavelength λ 1 =633 nm, a phase step of Δ ϕ 1 =14.055=4.47 π was obtained, which is equivalent to a phase step of because integer multiples of 2 π in phase cannot be distinguished. Thus, virtual wave vectors of about a quarter of the total bandwidth of the image could be generated for both wavelengths, providing best spatial resolution in the reconstructed amplitude and phase images. We note that for certain combinations of wavelengths, this situation might not be achievable and a virtual wave vector significantly smaller or larger than the quarter bandwidth might need to be accepted for one of the two wavelengths, resulting in a reduction of the spatial resolution in the reconstructed images for this wavelength. Comparison of SOH with interferometric methods The experiments shown in Fig. 6 were conducted under the same conditions to allow for a direct comparison between the different detection methods: same AFM tip, same tip illumination at 6 mW laser power, same tapping amplitude of 150 nm, same demodulation order n =3. The only difference is that two different piezo stages have been used for implementing a phase modulation of the reference wave. In case of Fig. 6b (quadrature), where fast mirror switching was required, and in case of Fig. 6c,e (pseudoheterodyne), where fast mirror vibration was required, we used a linear piezo stage with 100 μm travel (Physikinstrumente, model P-611). In case of Fig. 6d (SOH), a linear piezo stage with 800 μm travel (Physikinstrumente, model PiHera PI-628) was employed. In Fig. 6a,b,d , the detector signal was recorded with a fast data acquisition card and demodulation was performed on a computer using an integration time of 0.19 ms per pixel. In Fig. 6c,e , a commercial PSH detection module (Neaspec PMDK-2) was employed for signal demodulation, where the minimum integration time is 6.5 ms per pixel. Map of grain boundaries in CVD-grown graphene The infrared amplitude and phase images in Fig. 4c,d in the main text show a network of lines in the graphene sample, revealing both the graphene grain boundaries and the graphene wrinkles. The graphene wrinkles appear as long straight lines with lengths of several micrometres. Furthermore, graphene wrinkles appear as bright lines in the topography image in Fig. 4a with a typical height of 4 nm. In contrast, graphene boundaries form closed paths and usually three lines join in one point. Moreover, graphene boundaries are barely visible in the topography image, appearing as faint lines with a typical height of 1 nm because they are often decorated by contaminations (see also the zooms in Fig. 4e ). In the following, it will be described how the map of grain boundaries shown as black lines in Fig. 4f was derived. As a first step, a map of all lines was derived manually from the infrared amplitude and phase images in Fig. 4c,d . Then, this map was superposed with topography and lines previously identified as graphene wrinkles because of their height were removed from the map. After this step, a few straight lines remained that did not have the structure of grain boundaries and were thus removed manually. Samples The antenna sample was fabricated by electron-beam lithography on a CaF 2 substrate and has been analysed and described in ref. 65 . The graphene was grown in a CVD process on Cu and transferred to a 300-nm SiO 2 layer on a Si substrate. How to cite this article: Schnell, M. et al . Synthetic optical holography for rapid nanoimaging. Nat. Commun. 5:3499 doi: 10.1038/ncomms4499 (2014).